Quantum-to-continuum prediction of ductility loss in aluminium–magnesium alloys due to dynamic strain aging Negative strain-rate sensitivity due to dynamic strain aging in Aluminium–5XXX alloys leads to reduced ductility and plastic instabilities at room temperature, inhibiting application of these alloys in many forming processes. Here a hierarchical multiscale model is presented that uses (i) quantum and atomic information on solute energies and motion around a dislocation core, (ii) dislocation models to predict the effects of solutes on dislocation motion through a dislocation forest, (iii) a thermo-kinetic constitutive model that faithfully includes the atomistic and dislocation scale mechanisms and (iv) a finite-element implementation, to predict the ductility as a function of temperature and strain rate in AA5182. The model, which contains no significant adjustable parameters, predicts the observed steep drop in ductility at room temperature, which can be directly attributed to the atomistic aging mechanism. On the basis of quantum inputs, this multiscale theory can be used in the future to design new alloys with higher ductility. One major goal of computational material science, in the realm of mechanical properties of materials, is the parameter-free prediction of macroscopic failure of a metal at experimental size (mm to cm) and time (seconds) scales. Although it is clear that the collective behaviour of dislocations and their interactions with other defects (for example, solutes, grain boundaries, cracks) ultimately determines macroscopic failure, a direct connection between atomic scale phenomena and their macroscale consequences on failure has remained largely unsolved. In many applications such as metal-forming, the usable ductility of the material is limited by the onset of necking due to plastic instability. In the Al–5XXX alloys, a key class of lightweight metal alloys used in the automotive industry, the ductility shows a distinct drop around room temperature, being much larger at both lower and higher temperatures [1] . Reduced ductility is usually accompanied by unstable plastic flow with rapid local strain rate fluctuations, called Portevin Le-Chatelier (PLC) instabilities, which are manifested as serrations in the stress–strain curve [2] , [3] . Together, ductility loss and PLC effects limit the ability to form these materials into complex shapes under acceptable industrial conditions, and represent an impediment to wider application of these light alloys. Overcoming the low ductility, while maintaining the many desirable properties of these alloys, thus has tremendous practical consequences. More broadly, this problem is a case study for showing how rigorously developed multiscale models can connect observed macroscopic behaviour to underlying atomic and dislocation-level mechanisms. At the macroscopic continuum scale, ductility is known to be related to the work-hardening rate and the strain-rate sensitivity. A standard constitutive law for the flow stress as a function of the plastic strain and plastic strain rate of the form , where N is the strain hardening exponent and m is the strain-rate sensitivity, has been used to show that ductility limited by necking is highly sensitive to both N and m (ref. 4 ). Strain hardening is fairly well understood as being due to dislocation multiplication and the formation of an increasingly dense network of dislocation junctions [5] . Strain-rate sensitivity is due, in general, to stress-driven thermally activated phenomena having diverse origins, including dislocation climb, grain boundary sliding and solute-drag phenomena, which control strain-rate sensitivity at high homologous temperatures, and thermally activated escape of dislocations from pinning obstacles, which dominate at low homologous temperatures [5] , [6] . In Al–5XXX alloys, the phenomenon of dynamic strain aging (DSA) actually renders the steady-state strain-rate sensitivity negative, that is, m <0 (refs 1 , 7 ). Moreover, in such aging materials, the onset of instabilities is governed by the full dynamic, non-steady-state response of the material [8] , [9] , [10] , [11] , and so the problem is even richer and more complex than in materials with m >0. There have been many phenomenological approaches where the DSA behaviour is introduced by fiat [9] , [10] , [12] and then model parameters are fit to particular material data set. While such approaches reproduce instabilities, because m <0 is built into the models, and can be used to model some aspects of macroscopic structural response in the DSA regime using parameters calibrated with experimental data, they reveal little about the true underlying material dependence of the macroscopic behaviour. Thus, there is a continued need for deeper understanding and real predictive power. Here, we present a hierarchical multiscale mode that faithfully carries nano- and microscale information up to the macroscale, leading to quantitative prediction of ductility as a function of the alloy chemistry and test conditions, and providing a framework for the design of new materials with improved performance. A schematic of the overall flow of the quantum-to-continuum multiscale model is shown in Fig. 1 . The solute strengthening and the aging process are related to the energetics of solute atoms in the dislocation core as computed by quantum mechanics ( Fig. 1a ). The aging process occurs by ‘cross-core’ diffusion of solutes. This aging process affects the strengthening of mobile dislocations in two ways: by cross-core diffusion along the mobile dislocation and by cross-core diffusion along the forest dislocations ( Fig. 1b ). These two processes are then combined into an overall energy barrier for the thermally activated escape of a mobile dislocation from its current pinned site, which determines the frequency of dislocation escape events ( Fig. 1c ). The time-dependent energy barrier is then used in a full kinetic model that accounts for the aging histories of the entire collection of mobile dislocations in the volume, leading to a new constitutive model for the plastic strain rate as a function of the underlying material properties, the loading and the temperature ( Fig. 1d ). This new constitutive model is used within a commercial finite-element code to predict the deformation of test specimens identical to those used in experiments, including the rate sensitivity and temperature dependence of the ductility ( Fig. 1e ). A reduction of ductility around room temperature and the occurrence of PLC-type instabilities are predicted by the model, with the ductility in quantitative agreement with experiments. The full model then allows for ductility to be predicted as a function of changes in the alloy composition. Furthermore, these predictions are obtained only with the use of the precise quantum solute energetics and the detailed forms of the energy barriers incorporated into the derived constitutive model. The use of semi-empirical potentials for atomic energies, of standard energy barrier models, of ad hoc Kocks–Mecking-type forest-rate sensitivity, or of other often-used phenomenological constitutive models, leads to results that do not predict the correct ductility, rate sensitivity versus temperature, or PLC-type behaviour. 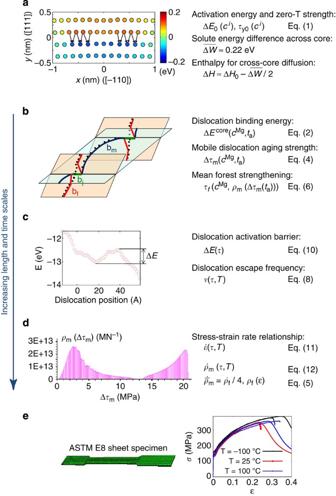Figure 1: Overview of the multiscale dynamic strain aging model. Schematic overview of the hierarchical multiscale model for dynamic strain aging in Al–Mg alloys. The relevant physical quantities computed at each level are listed, which are functions of the primary variables shown as well as other parameters computed at lower scales. (a) Solute strengthening and aging, (b) mobile and forest strengthening, (c) thermally activated dislocation motion, (d) continuum constitutive model and (e) ductility predictions.ciis the concentration of solutei,tais the aging time of a mobile dislocation,ρm(Δτm(ta)) is the mobile dislocation density distribution function,τis the macroscopic flow stress,εis the strain,is the strain rate andTis the absolute temperature. Figure 1: Overview of the multiscale dynamic strain aging model. Schematic overview of the hierarchical multiscale model for dynamic strain aging in Al–Mg alloys. The relevant physical quantities computed at each level are listed, which are functions of the primary variables shown as well as other parameters computed at lower scales. ( a ) Solute strengthening and aging, ( b ) mobile and forest strengthening, ( c ) thermally activated dislocation motion, ( d ) continuum constitutive model and ( e ) ductility predictions. c i is the concentration of solute i , t a is the aging time of a mobile dislocation, ρ m (Δ τ m ( t a )) is the mobile dislocation density distribution function, τ is the macroscopic flow stress, ε is the strain, is the strain rate and T is the absolute temperature. Full size image Model summary We now present the details of the model, starting at the bottom by looking at the quantum scale that defines solute dislocation interaction energies. Figure 1a shows the interaction energy of a substitutional Mg solute in the core of an Al edge dislocation for all positions around the core. From these energies, and similar ones for other solutes, the rate-dependent solute strengthening is controlled by a fundamental energy Δ E 0 and zero-temperature strength τ y 0 for solute strengthening computed as in refs 13 , 14 where c i , and denote the solute concentration (atomic fraction), energy barrier and zero-temperature strength for each solute element i in the alloy, given in ref. 14 . Dynamic strain aging occurs by migration, via a single vacancy-mediated hop, of the Mg solutes on the first row of atoms on the compression side to the first row of atoms on the tension side in the cores of the partial dislocations in the dissociated core, as indicated in Fig. 1a . Along the width of the dissociated quantum core ( b =dislocation Burgers vector), the average net energy gain per solute in moving from the compression to the tension side is . Note that these values for and , being obtained from ab initio simulations, are the best estimates using the state-of-the-art methods [14] and differ from earlier estimates obtained using semi-empirical potentials [15] . The energy barrier for the diffusive hop across the core in the regions of the two partial dislocations is , where the value of Δ H 0 (=0.97 eV) is computed using the Liu et al. [16] EAM potential for the Al–Mg system, which predicts the bulk diffusion migration barrier very well [17] . The ‘cross-core’ diffusion, occurring over an aging time t a , increases the binding energy of that dislocation to its current position as in ref. 15 where is the characteristic cross-core diffusion time, ν 0 is a fundamental attempt frequency, c Mg is the average concentration of Mg solute atoms, β =8/9 is the fraction of core sites providing solutes ( Fig. 1a ), k is Boltzmann’s constant, and T is the absolute temperature. Cross-core diffusion influences both the strength of the mobile dislocations and the forest strengthening arising when the mobile dislocations form junctions with dislocations on other slip systems ( Fig. 1b ). The mobile strengthening of an individual dislocation is directly proportional to the rate of change of core energy with respect to the dislocation position, and has been derived as in ref. 15 , which serves to define Δ τ max . The parameter α depends on how the energy of the dislocation changes as it attempts to glide away from the diffused solutes under an applied stress, and for the energies in Fig. 1a is α =0.54. The aging times of the collection of mobile dislocations are statistically distributed, as mobile dislocations become pinned and then unpinned by thermal activation. Using equation (4), we can characterize the distribution of aging times by a corresponding distribution of the mobile density ρ m (Δ τ m ), for 0<Δ τ m <Δ τ max , such that ρ m (Δ τ m )dΔ τ m is the density of mobile dislocations having aging strengths within an interval dΔ τ m around Δ τ m (ref. 18 ). Forest strengthening in the absence of aging is associated with the evolution of forest dislocation density in the material as where ρ f is the forest density, is the line tension energy per unit length of dislocation, G is the shear modulus, ν is the Poisson ratio, and the numerical coefficient 1.37 is an average over FCC junction types. The work hardening due to dislocation multiplication and annihilation processes has no direct connection to the dynamic strain aging phenomenon and so we use a Voce law for the forest dislocation density evolution, given by The saturation dislocation density and reference plastic strain ε sat are used as fitting parameters for the work hardening at low temperature where dynamic strain aging effects are negligible. With being fit, the precise prefactors in the expression for are not important. For the assumed multi-slip conditions, we take the total mobile density on any one slip system to be . This assumption is consistent with a Taylor model for an FCC polycrystal, where five slip systems are active in any grain with the dislocations on any given slip system interacting with forest dislocations on four other slip systems. More detailed phenomenological treatments of dislocation multiplication exist where the forest and mobile dislocation densities can evolve independently [19] . However, the simple two parameter model of equation (5) provides a good fit to the experimental stress–strain curve at low temperatures (see below). Implementation of a more-detailed model would not provide significantly better results at the stress–strain level but might have some influence on more subtle features; this is beyond the scope of the present work. The additional forest strengthening due to cross-core diffusion is directly proportional to Δ E core because, in forming a junction with the mobile dislocation, the forest dislocations must be peeled away from the energetically favourable positions created by solute cross-core diffusion along the forest dislocations before the formation of the junction [20] , [21] ( Fig. 1b ). The total forest strengthening, if all the forest dislocations were aged over the same time t af , is thus where the factor of 8.7 emerges from averaging over FCC junction types [22] . In multi-slip conditions, the dislocations on one slip system serve as the forests for dislocations on other slip systems. Therefore, the forest strengthening of a mobile dislocation is due to its interaction with an array of forest dislocations that have the same distribution of aging times as the mobile dislocations and hence a distribution of junction strengths. The average strengthening of a dislocation encountering an array of forest dislocations with different junction strengths (due to different aging times) is the root-mean-square of the individual strengths [23] , [24] . Thus, we can write the forest strengthening in terms of the distribution of mobile strengths as Motion of a mobile dislocation proceeds by thermal activation over an energy barrier ( Fig. 1c ), with the rate of escape of a dislocation that has been pinned for time t a following the Arrhenius behaviour The stress- and time-dependent energy barrier in equation (8) is determined by (i) the barrier for solute strengthening due to solute atoms without any cross-core diffusion (equation (1)), (ii) the backstress due to the mobile aging associated with cross-core diffusion (equation (4)) and (iii) the backstress due to forest strengthening with aging (equations (6) and (7)). The energy barrier as a function of the applied stress at any time t is taken as Equation (9) is consistent with an additive strengthening by solutes and forest dislocations usually assumed at finite temperatures. The presence of the forest hardening term in the denominator of equation (9) is justified by analysis of the Haasen plot behaviour of a range of binary Al–X alloys [25] . At the temperatures of interest here (T~300 K), additional long-range contributions to the solute-strengthening energy barrier arise such that the appropriate model is the modified form ref. 14 The macroscopic plastic strain rate is the net rate of motion of all the mobile dislocations as they unpin, move and become pinned again by forest dislocations and solutes, with cross-core diffusion in the mobile dislocations starting upon each new pinning event. At any time t , the strain rate is given by the rate at which the statistical collection of mobile dislocations can escape over their barriers, which can be written in terms of the mobile age distribution function ρ m (Δ τ m ) as in ref. 18 where the second term represents the additional (small) contribution from the nucleation of new mobile dislocations that follows from the Voce law (equation (5)) and . Figure 1d shows a typical shape of the mobile density distribution function ρ m (Δ τ m ) in the aging regime of strain rates and temperature. Furthermore, the time evolution of ρ m (Δ τ m ) is given in terms of the partial differential equation with and denoting the derivative of equation (4) with t a (ref. 18 ). To connect the shear stress τ to an applied tensile stress σ, we use a Taylor factor, σ = Mτ with M =3.0 appropriate for untextured polycrystals. The new and crucial features in the present formulation are as follows: (i) the use of the quantum-computed dislocation structure and solute/dislocation interaction energies for the underlying solute strengthening and cross-core aging parameters, which also enables future material design, (ii) the recognition that the forest and mobile aging times are the same on average, leading to equation (7), (iii) the introduction of the forest strengthening term in the denominator of the energy barrier of equation (9) motivated by experimental data, (iv) the use of the standard Voce law of equation (5) to conform with established work-hardening models and (iv) the integration of the entire set of models into a single hierarchical framework with the computationally feasible constitutive model of equations (11) and (12). All of these new features are essential for making quantitative predictions of ductility. Tensile behaviour of AA5182–O alloy Detailed results on the strain-rate sensitivity and ductility of test coupons as a function of temperature in AA5182–O (composition (wt. %): Mg 4.5%, Cr 0.1%, Si 0.2%, Cu 0.15%, Mn 0.3–0.5%, Fe 0.35%, Zn 0.25%, Ti 0.1%) have been published by Picu et al. [1] Equation (1) is used to predict the solid solution strengthening parameters Δ E 0 and τ y0 . The concentration of Fe in solid solution is difficult to determine and is the one element for which the ab initio calculations do not match the experiment. We therefore use the apparent values of and back calculated from experiments [13] , [14] , and treat c Fe as an adjustable parameter to match the initial experimental yield stress in the nonaging regime at T =−100 °C and strain rate 10 −3 s −1 . The two forest density evolution parameters ρ f sat and ε sat are then used to fit the experimental stress–strain curve after yielding only at T =−100 °C and , conditions under which there are no aging effects. These three fitted parameters take the values c Fe =0.035%, ρ f sat =12.3 × 10 14 m −2 and ε sat =0.39; all other material properties are computed from the quantum, atomistic or dislocation models and their values are given in Table 1 . Table 1 Model parameters for aluminium. Full size table We first use the model to predict the strain-rate sensitivity parameter m . Picu et al. [1] measured the steady-state stresses σ 1 and σ 2 at a given plastic strain at two values of the strain rate and , with , to obtain m as . The instantaneous strain-rate sensitivity m i , which must always be positive, was measured using strain-rate jump tests between the same strain rates. We predict m and m i using the same procedures but with numerical tests. The measured and predicted values for m between the strain rates and as a function of plastic strain and at various temperatures are shown in Fig. 2 . The model correctly predicts negative rate sensitivity at 25 and 50 °C, and positive rate sensitivity at 110 °C and increasing with plastic strain. The general dependence of m on plastic strain demonstrates the crucial role of aging on the forest strengthening. The instantaneous strain-rate sensitivity m i is also shown in Fig. 2 , and the predictions again agree with experiments including the increase in m i with increasing plastic strain. The model does not match the experiments perfectly, but there are no adjustable parameters, the difference of roughly 25 °C in the temperature dependence is below the accuracy of the energetics used in the model, and the model captures the crucial phenomenon of m <0 in magnitude and temperature range. The predictions at 110 °C are slightly lower than experiments, possibly indicating the onset of additional high temperature mechanisms, such as solute drag that are not in the current model. Figure 3 shows the steady-state rate sensitivity m at 10% plastic strain between the strain rates and as a function of temperature. 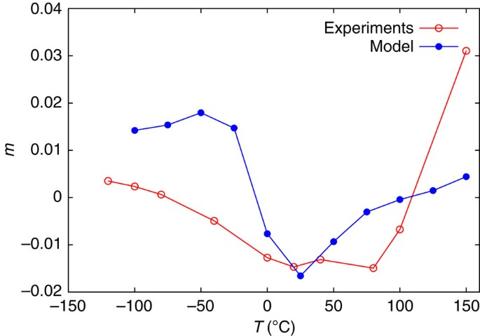Figure 3: Strain rate sensitivity as a function of temperature. Steady-state rate sensitivity parametermmeasured at 10% plastic strain between the strain ratesandas a function of the test temperature. Again, the model predictions for m are seen to be in good agreement with the experimental data in magnitude and sign, even though the domain of negative strain-rate sensitivity is somewhat narrower than in the experiments. 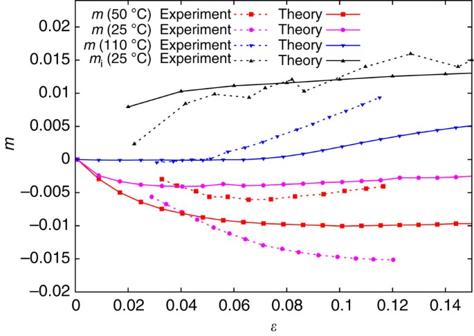Good parameter-free predictions of the strain-rate sensitivity are the first main result of this paper. Figure 2: Evolution of strain rate sensitivity with plastic strain. Steady-state rate sensitivity parametermand instantaneous rate sensitivity parametermibetween the strain ratesandversus plastic strain, at various temperatures. Figure 2: Evolution of strain rate sensitivity with plastic strain. Steady-state rate sensitivity parameter m and instantaneous rate sensitivity parameter m i between the strain rates and versus plastic strain, at various temperatures. Full size image Figure 3: Strain rate sensitivity as a function of temperature. Steady-state rate sensitivity parameter m measured at 10% plastic strain between the strain rates and as a function of the test temperature. Full size image We now apply the model to predict ductility of laboratory tensile coupons as a function of temperature using full three-dimensional explicit dynamic finite-element simulations to capture possible dynamic instabilities. The constitutive model is implemented in the commercial code Abaqus via a user-defined material subroutine. We created models corresponding to those studied by Picu et al. , [1] that is, 1 mm-thick rolled and annealed sheets fabricated into ASTM-E8 specimens (inset of Fig. 4 ), and performed computational tensile tests. We define ductility as the strain at the onset of localization (necking). As the onset of localization in real specimens is always sensitive to small defects in the specimen geometry, such as the thickness for sheet metals, we introduce a smooth thickness variation of 0.1% of the nominal thickness through the sample gauge section, with the thinnest cross-section at the centre of the specimen. This ‘defect’ size is chosen to reproduce the measured ductility at low temperatures below the regime where dynamic strain aging affects the ductility (cf. Fig. 5 ). 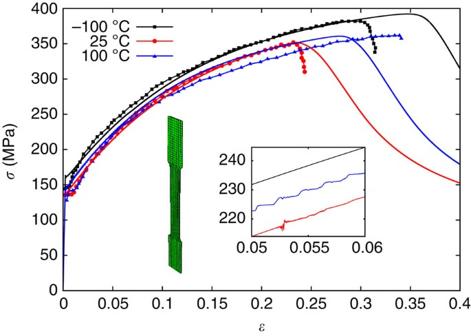Figure 4: Stress–strain curves for AA5182 tensile specimens. True stress versus true strain response of AA5182, as measured1(discrete points) and as predicted (lines). Inset: sample shape and mesh for ASTM-E8 specimen. Inset: magnified portion of the predicted stress–strain curves showing oscillations due to plastic flow instabilities. Figure 4 shows the true stress versus logarithmic strain within the specimen gauge section predicted by the model and as measured at T =−100, 25 and 100 °C at a nominal applied strain rate of 10 −3 s −1 . The true stress is the force per unit current cross-sectional area assuming that the deformation is homogeneous within the gauge section and hence results beyond the onset of necking are not representative of the true material response; the strain at the onset of necking is henceforth defined as the ductility. The model predicts that the ductility is lowest at room temperature, in good agreement with the experiments. The predicted temperature sensitivity of the flow stress is also in agreement with the experiments. Figure 4: Stress–strain curves for AA5182 tensile specimens. True stress versus true strain response of AA5182, as measured [1] (discrete points) and as predicted (lines). Inset: sample shape and mesh for ASTM-E8 specimen. Inset: magnified portion of the predicted stress–strain curves showing oscillations due to plastic flow instabilities. 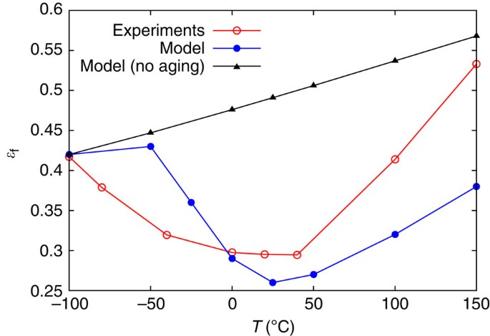Figure 5: Comparison of ductility predictions with experiments. Tensile ductilityεfas a function of temperatureT, as measured in experiments of Picuet al.1(red curve) and as computed by the present multiscale model with dynamic strain aging (blue curve). Also shown is the model prediction of ductility in the absence of dynamic strain aging (black curve), demonstrating that the observed ductility loss is due to the dynamic strain aging. Full size image Figure 5: Comparison of ductility predictions with experiments. Tensile ductility ε f as a function of temperature T , as measured in experiments of Picu et al. [1] (red curve) and as computed by the present multiscale model with dynamic strain aging (blue curve). Also shown is the model prediction of ductility in the absence of dynamic strain aging (black curve), demonstrating that the observed ductility loss is due to the dynamic strain aging. Full size image Figure 5 shows the ductility versus temperature as predicted and the experimentally measured total elongation at failure. As the post-localization behaviour and material separation are not captured in the simulations, the failure strains reported are the engineering strains corresponding to the maximum value of true stress attained in the simulations. However, as experimental data indicates that the onset of localization is quickly followed by complete specimen failure in these alloys, comparison of trends between the two measures is reasonable. The model correctly predicts the ductility minimum observed around room temperature and also the magnitude of the drop in ductility. For comparison, the predicted ductility as a function of temperature in the absence of DSA is also shown in Fig. 5 (achieved by setting the cross-core diffusion energy barrier to a very high value), and shows a monotonic increase with temperature, thus establishing that the DSA and associated negative strain-rate sensitivity are the mechanistic drivers of the loss of ductility. As the effects of higher temperature or lower strain rate are equivalent in the theory of thermally activated dislocation glide, the existence of a ductility minimum temperature at fixed strain rate implies that a similar minimum ductility strain rate must exist at a fixed temperature. 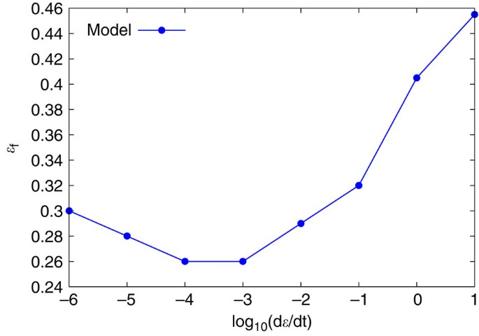Figure 6: Ductility as a function of strain rate. Tensile ductilityεf, defined as the strain corresponding to the maximum true stress attained, as a function of the applied strain rate atT=25 °C. Figure 6 shows the failure strains at T =25 °C as a function of the strain rate and the lowest ductility is predicted at . The results in Figs 4 and 5 are remarkable in that the model contains no adjustable parameters relevant to the DSA phenomenon and is hence truly predictive. The good correspondence between the simulated and experimental variation of ductility with temperature is the second, and main, result of this paper. Figure 6: Ductility as a function of strain rate. Tensile ductility ε f , defined as the strain corresponding to the maximum true stress attained, as a function of the applied strain rate at T =25 °C. Full size image Closer inspection of the stress–strain curves in Fig. 4 reveals that at temperatures T =25–100 °C, the stress–strain curves exhibit small oscillations (inset, Fig. 4 ) that are accompanied by rapidly moving bands of high strain rate travelling up and down the specimen gauge section, similar to PLC bands. 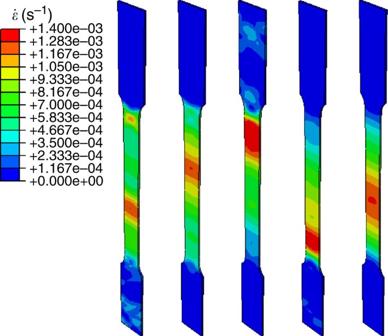Figure 7: Snapshots of high strain rate bands during serrated flow. Contours of the axial strain rate at subsequent time steps during theT=50 °C simulation, showing the travelling high strain rate bands during serrated flow. The average axial strain rate in the gauge section is. Figure 7 shows an example of the travelling bands observed in the simulations at T =50 °C in the form of a series of snapshots showing the contours of axial strain rate at subsequent instants of time. The occurrence of PLC bands is sensitive to the transient response following a step change in the strain rate [26] . In fact, our previous DSA model failed to yield instabilities precisely because the transient response was too slow [18] . 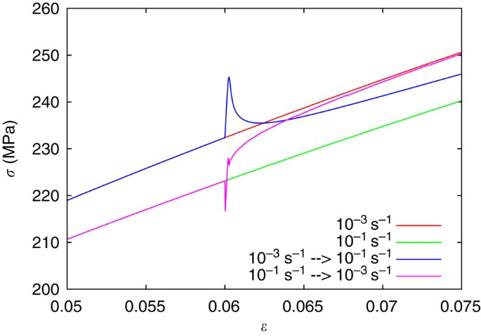Figure 8: Transient response of the model in the regime of negative strain rate sensitivity. Transient response of the DSA model for a step change in strain rate betweenandatT=50 °C andε=0.06. Only a portion of the stress–strain curve near the strain-rate step is shown. Figure 8 shows the predicted transient response following step changes in strain rate between and at ε =0.06 and T =50 °C (in the regime of negative strain-rate sensitivity). After the instantaneous stress jump associated with the positive instantaneous strain rate sensitivity, the transient relaxation to the steady-state rate sensitivity is quite fast, especially for a decrease in strain rate, and evidently fast enough to trigger the dynamic PLC-like instabilities. The emergence of PLC-like phenomena from the theory with no additional inputs is the third main result of this paper. Figure 7: Snapshots of high strain rate bands during serrated flow. Contours of the axial strain rate at subsequent time steps during the T =50 °C simulation, showing the travelling high strain rate bands during serrated flow. The average axial strain rate in the gauge section is . Full size image Figure 8: Transient response of the model in the regime of negative strain rate sensitivity. Transient response of the DSA model for a step change in strain rate between and at T =50 °C and ε =0.06. Only a portion of the stress–strain curve near the strain-rate step is shown. Full size image We have demonstrated that quantitative parameter-free predictions of complex macroscale material behaviour, ductility, can be achieved using rigorously developed multiscale models. The multiscale modelling approach establishes a direct connection between material chemistry, nanoscale mechanisms, mesoscale dislocation mechanics and macroscopic rate-dependent flow behaviour. Several comments are in order regarding the ductility predictions obtained using the DSA model. The results in Fig. 5 show that, although the model performs well over a wide range of practically important temperatures, −100 to 100 °C, the discrepancy with experiments appear to increase towards higher temperatures. This is to be expected since some phenomena such as solute drag, omitted in the present DSA model, are expected to contribute significantly to the rate sensitivity at higher temperatures. The material parameters for the Al–Mg system, computed from ab initio and atomistic simulations, are summarized in Table 1 . Among these parameters, the value of α , which is related to the change in solute dislocation interaction energy as a function of the dislocation position, is known with the least certainty. The value quoted in Table 1 is the best estimate for α based on a model of cross-core diffusion over 3/5 of the dissociated dislocation core width (region of fastest cross-core diffusion) with four atomic sites on the compression side feeding solutes into three sites on the tension side of the slip plane. Parameter sensitivity analysis for α , not reported here, reveals that α has an indirect effect on rate sensitivity at high T , with lower values of α yielding higher rate sensitivity and consequently higher ductility, closer to the experimental trends in ref. 1 . Although making good predictions of strain-rate sensitivity and ductility with no adjustable parameters, the model remains imperfect in predictions of the plastic instabilities (PLC effects) as experimentally observed serrations in the stress–strain curve are more pronounced than predicted. The model may thus still be lacking some physics relevant to the PLC phenomenon that does not otherwise influence steady-state rate-dependent response of the material. For instance, correlated depinning of aged dislocation ensembles due to long-range interactions has been postulated as a mechanism driving PLC. Hahner [27] and others proposed that ‘collective slip’ events are necessary to yield negative strain rate sensitivity, and hence PLC. However, subsequent work [21] , [22] culminating in our model here shows that negative rate sensitivity can emerge without such collective effects due to the combination of mobile and forest dislocation aging. Our predictions for the correct domains of negative strain-rate sensitivity and for the occurrence of travelling PLC-like bands show that our model, with no adjustable parameters and without invoking such collective/interaction effects, contains the transient dynamic response sufficient to predict PLC effects. Thus, collective effects are not necessary to obtain serrated flow. Nonetheless, collective or long-range effects may influence the detailed dynamics during instabilities and may be one mechanism by which the prediction of PLC phenomenon can be improved, relative to the present model. This is a suggested topic for future research. With a mechanistic and predictive multiscale model, we can embark on the path of virtual design of new alloys with improved macroscopic properties, such as ductility. Experimental collaborators are presently working on fabricating and testing new Al–Mg–X alloys that are predicted by the present multiscale model to have improved ductility; the results of this difficult task will be reported in the future. Finally, the accomplishment here of quantitatively predicting essentially all the complex, interacting dynamic phenomena occurring in one particular metal alloy, Al–Mg, provides the hard evidence that rigorous multiscale modelling can yield new and valuable insights into scientifically interesting and technologically valuable material behaviour. How to cite this article: Keralavarma, S. M. et al. Quantum-to-continuum prediction of ductility loss in aluminium–magnesium alloys due to dynamic strain aging. Nat. Commun. 5:4604 doi: 10.1038/ncomms5604 (2014).